Non-reciprocal and highly nonlinear active acoustic metamaterials Unidirectional devices that pass acoustic energy in only one direction have numerous applications and, consequently, have recently received significant attention. However, for most practical applications that require unidirectionality at audio and low frequencies, subwavelength implementations capable of the necessary time-reversal symmetry breaking remain elusive. Here we describe a design approach based on metamaterial techniques that provides highly subwavelength and strongly non-reciprocal devices. We demonstrate this approach by designing and experimentally characterizing a non-reciprocal active acoustic metamaterial unit cell composed of a single piezoelectric membrane augmented by a nonlinear electronic circuit, and sandwiched between Helmholtz cavities tuned to different frequencies. The design is thinner than a tenth of a wavelength, yet it has an isolation factor of >10 dB. The design method generates relatively broadband unidirectional devices and is a good candidate for numerous acoustic applications. The development of acoustic metamaterials has brought with it a strong drive towards bringing electromagnetic concepts to acoustics. Thus, the extended range of material parameters provided by metamaterials has lead to the implementation of devices such as acoustic lenses [1] , [2] , [3] , [4] , [5] , [6] , or even exotic structures designed using coordinate transformation methods [7] , [8] . Recently, significant attention has been given to unidirectional devices that pass acoustic energy in only one direction [9] , [10] , [11] , [12] , [13] , [14] , [15] and therefore mimic the general behaviour of diodes in the microwave regime, and Faraday rotator media in the optical domain. The unidirectional acoustic devices are the focus of this article. These devices have received many names, such as acoustic diodes, rectifiers, isolators and non-reciprocal media. There is an on-going debate on what constitutes proper terminology. In this article, we take the more conservative approach of Maznev et al . [16] and only consider non-reciprocal media capable of breaking the transmission symmetry property, that is, they transmit acoustic energy in only one direction regardless of the spatial spectrum of the incident acoustic excitation. In other words, we eliminate passive devices [9] , [10] , [11] , [12] , [13] that exhibit time-reversal symmetry. The non-reciprocal devices fitting the above description reported so far [14] , [15] achieve non-reciprocity in nonlinear macroscopic structures that contain, among other elements, at least one phononic crystal filter. The idea behind this type of approach was adapted first in theory [17] from a thermal diode design [18] , [19] , [20] in which the heat transport due to phonons was controlled in a nonlinear, asymmetric structure (see Li et al . [21] for more details). The effectiveness of the acoustic non-reciprocal device strongly depends on the phononic filter selectivity, and, consequently, depends on the thickness of the phononic crystal, which necessarily needs to be much larger than the wavelength of the incoming acoustic wave. For example, Liang et al . [14] used a thickness of ≈30 λ, and Boechler et al . [15] employed a thickness of ≈10 λ, which makes these devices inadequate for audio and low-frequency applications. Instead, compact and subwavelength implementations are desirable in most practical applications. Metamaterial concepts have been shown to provide the right platform for the design of non-reciprocal electromagnetic media [22] . In this article, we non-trivially extend this methodology to acoustics, and describe a design approach that results in structures highly subwavelength, but strongly non-reciprocal for their size. We demonstrate this approach by designing a non-reciprocal device λ/10 thick and having an isolation factor of >10 dB. We use two highly subwavelength Helmholtz cavities tuned on different frequencies to create the asymmetry needed for the non-reciprocal behaviour. These cavities share a common wall consisting of a piezoelectric membrane (PZM) augmented by a nonlinear electronic circuit that sets the behaviour of the membrane. Similar to conventional acoustic media that absorb the incident sound field and then re-radiate it, the role of the membrane is to sense the ambient acoustic field and, at the same time, generate an acoustic response controlled by the electronic circuit. The Helmholtz cavities play the secondary role of matching the PZM impedance with that of the air background, thus increasing the intensity of the PZM acoustic response. Note that this approach complements the linear and reciprocal active architecture of Popa et al . [23] , which employed separate sensing and driven elements connected by linear circuits. Unlike previous designs that relied on very selective, therefore, bulky filters, the highly subwavelength Helmholtz cavities have a rather wide half-amplitude bandwidth of ≈40%. Instead, their key property is their improved directivity as sound sensors and generators, because they mostly couple to sound coming from the semiplane to which the cavity opening points. This design approach results in acoustically thin non-reciprocal structures having high isolation factors. The structures have relatively large bandwidths and are designed to be very robust given that the nonlinear behaviour is generated by the electronics and not by the physical structure of the material. 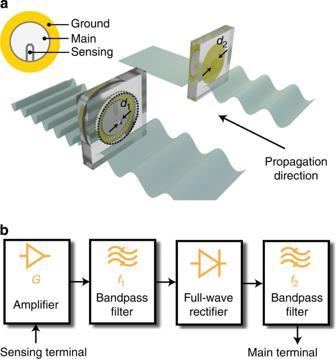Figure 1:Design and behaviour of the non-reciprocal active acoustic unit cell. (a) In one orientation (foreground) the cell passes acoustic energy, in the other (background) it blocks it. The cell is composed of the PZM shown in the inset sandwiched between two asymmetric Helmholtz cavities. One cavity is highlighted with dotted lines. The asymmetry is given by different diameters of the cavities openings (d1andd2). Inset: the PZM has three terminals and is used as both the sensing and driven element simultaneously. (b) Nonlinear electronic circuit driving the PZM. Non-reciprocal metamaterial cell design Figure 1a shows the non-reciprocal metamaterial cell representation (front and back) and behaviour. Central to the design is the PZM produced by Murata (part number 7BB-35-3CL0) and illustrated in the top-left inset. As with most commercial PZMs, a thin layer of piezoelectric ceramic is deposited on a brass disk. Two conducting electrodes are then deposited on top of the ceramic to create a two-capacitor, three-terminal membrane. This design, together with the property of the piezoelectric material to convert back and forth between electric and acoustic energy, allows us to use the membrane as an acoustic sensor of the background acoustic field and, at the same time, a sound-producing element able to change the acoustic properties of the incoming sound wave (spatial and temporal spectra) in the same way a conventional acoustic material functions. The small terminal forms the sensing terminal, while the big electrode covering most of the piezoelectric ceramic is called the main terminal. These terminals are connected to the electronic circuit whose block diagram is presented in Fig. 1b . The goal of the circuit is to double the frequency of the input signal centred around f 1 =1,500 Hz and is designed to have a 3-dB bandwidth of 20%. Figure 1: Design and behaviour of the non-reciprocal active acoustic unit cell . ( a ) In one orientation (foreground) the cell passes acoustic energy, in the other (background) it blocks it. The cell is composed of the PZM shown in the inset sandwiched between two asymmetric Helmholtz cavities. One cavity is highlighted with dotted lines. The asymmetry is given by different diameters of the cavities openings ( d 1 and d 2 ). Inset: the PZM has three terminals and is used as both the sensing and driven element simultaneously. ( b ) Nonlinear electronic circuit driving the PZM. Full size image More specifically, the sensed signal proportional to the external acoustic field is amplified in a one-stage pre-amplifier of gain G =140 implemented with the Texas Instruments OP37G operational amplifier (op-amp). The resulting signal is filtered with a two-pole bandpass filter tuned on frequency f 1 =1,500 Hz, having a 3-dB bandwidth of 300 Hz, and implemented with an OP27G op-amp in a standard Sallen–Key configuration. The next stage is a full-wave rectifier implemented for robustness with two OP27G op-amps. Finally, the output of the rectifier is filtered with a selective bandpass filter from WaveTek (model 852) tuned on f 2 =2 f 1 =3,000 Hz and having a bandwidth of 600 Hz. As with any full-wave rectifier, its efficiency to convert energy from f 1 to f 2 is 18%. For the purpose of this demonstration, the electronic circuit was assembled on breadboard, however, this simple design could easily be implemented as a tiny surface-mount circuit. The PZM is better matched to the air background using two cylindrical Helmholtz cavities of diameter D =33 mm. For clarity, the boundaries of one of the cavities are highlighted in Fig. 1a with dotted lines. The PZM is a common wall for both cavities. The height of each cavity is h =3.2 mm. The asymmetry in the two cavity geometries is given by the different opening sizes of diameters d 1 and d 2 drilled in the walls of thickness t =1.6 mm opposite to the PZM. The diameters d 1 and d 2 were computed to make the cavities resonate at frequencies f 1 and f 2 , respectively, by inverting the design formula provided by the PZM manufacturer in its applications manual, namely , where i ∈ {1,2}, f 0 i are the two cavities resonant frequencies and c 0 =343 m s −1 is the speed of sound in air. Using this equation we find that d 1 =3 mm provides a resonant frequency f 01 =1,472 Hz and d 2 =9 mm provides a resonant frequency of f 02 =3,049 Hz, which are close to the desired f 1 =1,500 Hz and f 2 =3,000 Hz. With these dimensions, the cell thickness is ~1 cm, and its transverse dimensions are 5 cm by 5 cm. As mentioned above, the key property of the Helmholtz cavities that enables the non-reciprocal behaviour is their directivity pattern. Thus, a wave at 1,500 Hz incident on the unit cell wall having the d 1 opening (foreground in Fig. 1a ) will couple strongly to the 1,500-Hz cavity, the electronic circuit amplifies and converts the signal to 3,000 Hz and the PZM converts it back to acoustic energy launched by the 3,000-Hz cavity in the semiplane in contact with its opening. The PZM essentially acts as a strong second harmonic generator. We call this orientation in which sound energy is produced in the direction of the transmitted wave the forward orientation. On the other hand, when the incident wave impinges from the opposite direction (background in Fig. 1a ), the wave couples very little with the 3,000-Hz cavity facing the direction of incidence. It couples even less so to the 1,500-Hz cavity because its opening is facing the opposite direction. As a result, the sensed signal will be greatly attenuated compared with the forward orientation. In addition, the thus diminished acoustic wave created by the PZM is launched back in the direction from which the incident wave arrived, because the opening of the 3,000-Hz cavity faces this latter direction. We call this the reverse orientation. The result is a highly non-reciprocal device. As with any active circuit, potential instability has to be taken into account owing to unavoidable feedback between the sensing and driven elements, which in this case are on the same PZM. In a linear circuit, the instability can be removed using S -parameter techniques [23] . The design presented in this article, however, is nonlinear, but feedback is much easier to control, as follows. The electronic circuits input and output signals are centred on different frequencies. The bandpass filters and their selectivity are judiciously chosen to counteract the high gain of the circuit pre-amplifier and essentially remove the feedback. More specifically, the filters are chosen such that their combined attenuation is bigger than the pre-amplifier gain at all frequencies. A photograph of the fabricated unit cell is shown in Fig. 2 . The cell is built by stacking six sheets of transparent Plexiglas on top of each other, with the PZM glued in between the third and fourth sheets, that is, the middle of the structure. Each sheet is a square 5 cm by 5 cm and 1.6 mm thick. Disks of various diameters are removed from the centre of each sheet using a laser cutter. The diameters of the top most and bottom most cutout disks are d 1 and, respectively, d 2 . The cutout diameters of the four sheets in the middle are D . The sheets are then taped together to obtain the final unit cell. Wires connected to the PZM terminals leave the cell through small grooves cut in between the second and third sheets. 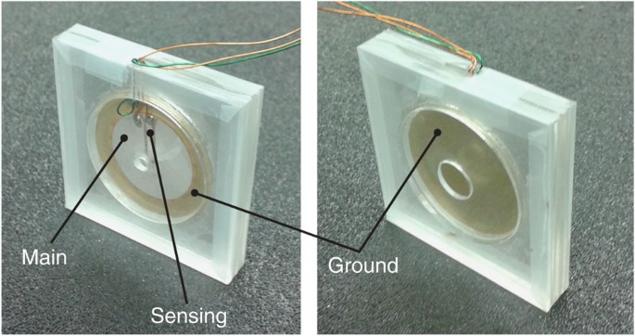Figure 2:Photograph of the fabricated unit cell. Left: the front side of the cell shows the three terminals of the PZM, and the Helmholtz cavity tuned on 1,500 Hz; right: the back side of the cell shows the Helmholtz cavity tuned on 3,000 Hz. The PZM is completely covered by the brass ground plane. Figure 2: Photograph of the fabricated unit cell . Left: the front side of the cell shows the three terminals of the PZM, and the Helmholtz cavity tuned on 1,500 Hz; right: the back side of the cell shows the Helmholtz cavity tuned on 3,000 Hz. The PZM is completely covered by the brass ground plane. 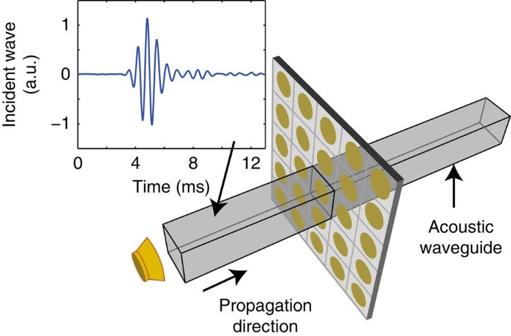Figure 3: Experimental set-up. Normal incidence on an infinite sheet of unit cells is mimicked experimentally by using a rectangular acoustic waveguide made of 5-mm thick rigid plastic and one unit cell placed in the middle of the waveguide. The waveguide is excited by a a speaker that sends a narrow, therefore, broadband pulse. The graph shows the measurement of the incident pulse. Full size image Measurements Figure 3 shows a possible way to deploy this unit cell as a sheet composed of multiple unit cells positioned in a rectangular lattice. We demonstrate this situation in an experiment. The set-up is simulated in the lab by using one unit cell placed in a rectangular waveguide, that is, a hollow rectangular pipe, having the same transverse dimensions as the cell and operated in a single-mode regime. Note that in this configuration the waveguide walls act as periodic boundary conditions. The waveguide is single mode for frequecies below f c =3,430 Hz, and, consequently, the device working frequencies were chosen such that f 1 < f 2 < f c . Figure 3: Experimental set-up. Normal incidence on an infinite sheet of unit cells is mimicked experimentally by using a rectangular acoustic waveguide made of 5-mm thick rigid plastic and one unit cell placed in the middle of the waveguide. The waveguide is excited by a a speaker that sends a narrow, therefore, broadband pulse. The graph shows the measurement of the incident pulse. Full size image Although this experimental set-up simulates normal incidence on an infinite sheet of metamaterial unit cells, the unidirectional metamaterial sheet would function well for most angles of incidence. This is because each Helmholtz cavity couples well to waves coming from the semiplane towards which the opening of the Helmholtz cavity faces for most wave directions. There is, however, a decrease in the coupling efficiency that may become an issue for steep angles of incidence bigger than ~70°, with 0° corresponding to normal incidence. A computer-controlled speaker launches a narrow Gaussian pulse centred on f 1 =1,500 Hz inside the waveguide. The pulse equation is given by p i ( t )= A exp(− at 2 )cos(2 πf 1 t ), where t represents the time in seconds, A is an arbitrary amplitude and a =1.66 × 10 6 s −2 . The time domain waveform measured by a microphone placed 60 cm in front of the cell is shown in the top-left corner of Fig. 3 . We note that the measured incident pulse width is ~3 ms and matches well with the above equation, except for the unavoidable phase shift introduced by the speaker and microphone and the small tail produced by the inertia of the speaker’s membrane typical in this type of systems. 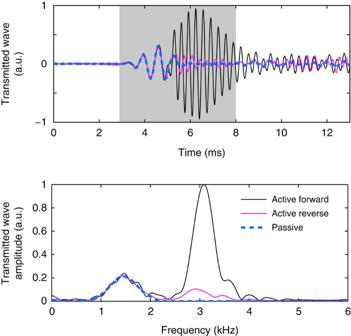Figure 4:Transmission measurements. Time (top) and frequency (bottom) measurements of the wave transmitted through the unit cell in three cases: cell unpowered (dashed line), cell powered in the forward, transparent orientation (solid black) and cell powered in the reverse, opaque orientation (solid light red). The grey shaded region represents the time window ΔTused to compute the isolation factorF. The measurements were repeated three times and each time the results were virtually identical. Figure 4 shows the time and frequency domain waveforms transmitted through the unit cell measured 40 cm behind it in three instances: the unpowered unit cell, the powered cell in the forward and reverse orientations. Figure 4: Transmission measurements . Time (top) and frequency (bottom) measurements of the wave transmitted through the unit cell in three cases: cell unpowered (dashed line), cell powered in the forward, transparent orientation (solid black) and cell powered in the reverse, opaque orientation (solid light red). The grey shaded region represents the time window Δ T used to compute the isolation factor F . The measurements were repeated three times and each time the results were virtually identical. Full size image With the unpowered structure (see the dashed blue curve), only a fraction of the incident acoustic energy is transmitted through the cell owing to its thickness being λ/20 at the incident wave frequency of 1,500 Hz. The energy transmitted through the powered cell positioned in the forward orientation is significantly increased due to the cell response at f 2 =3,000 Hz. The relatively broadband of the electronically enhanced PZM means that the shape of the transmitted pulse maintains the envelope of the incident wave, but the pulse frequency shifts to f 2 . The effect of the system bandwidth on the pulse spectra is evaluated from Fig. 4 (bottom). Thus, the 3-dB bandwidth of the second harmonic pulse would be 482 Hz, that is 16.1%, in an ideal system with infinite bandwidth. The second harmonic spectrum measured in the forward orientation has a bandwidth of 348 Hz, that is 11.6%, which confirms that the design is broadband. The powered cell positioned in the reverse orientation transmits very little energy and, therefore, behaves very similar to the unpowered cell in the transmission direction. The cell response due to the electronics, that is, the strong second harmonic produced by the PZM, is delayed by 2 ms compared with the passive response, that is, the energy transmitted at the fundamental frequency. The delay is almost entirely caused by the selective filters employed by the electronic circuit. More specifically, the bandpass filter before the rectifier in Fig. 1b delays the response by 0.38 ms, while the filter following the rectifier is responsible for 1.5 ms of the delay. This delay is suitable for the application described here, however, if desired, it can be further reduced using different electronic circuit designs. While the selectivity is needed to control the feedback between the input and output of the electronics, the delay can be shifted to frequencies outside the band of interest, for example, by using a combination of less selective bandpass filters and rejection band filters. To quantify the cell non-reciprocity, we define the isolation factor as the difference between the power transmitted in the forward and reverse orientations. The isolation factor in dB is expressed mathematically as , where p f and p r are the pressure fields measured in the forward and, respectively, reverse orientations, and Δ T =5 ms is the time interval containing the transmitted pulses, and illustrated in Fig. 4 as the grey area. The length of Δ T was chosen such that it contains the 2 ms delay of the active response and the first 3 ms of the active cell response, that is, the width of the incident pulse. Note that this conservative choice of Δ T leaves out the tail of the active response induced by the finite bandwidth of the cell and, therefore, underestimates F to some degree. Using this definition we obtain F =10 dB. The limiting factor of the design presented here is the energy transmitted through the highly subwavelength unit cell at the fundamental frequency f 1 even when the cell is unpowered. Note that the cell geometry is not resonant, therefore, this energy is lower bounded by the mass density law that states that the transmission coefficient is inversely proportional to the material thickness and mass density [24] . To see how big a limitation this is, we can define a second harmonic isolation factor, F 2 , that does not take into account the acoustic energy passing through the passive structure. More specifically, F 2 is defined similar to F , but derived based only on the second harmonic pressure fields at 3,000 Hz. We obtain in this case F 2 =19 dB, a testament of how non-reciprocal the design is. The cell electronics allow dynamically tunable cell properties. The isolation factors F and F 2 can be improved by increasing the amplifier gain G . This is achieved at the expense of higher isolation needed between the bands centred on the fundamental and second harmonics necessary to reduce the amplifier feedback. In turn, this leads to increased electronic circuit complexity. The phase through the electronic circuit is tunable as well, and it is an additional degree of freedom usable in some applications. For example, it can be used to implement unidirectional acoustic lenses by varying the phase delay through each cell in the same way reciprocal passive metamaterial lenses are designed [1] , [2] , [3] , [4] , [5] , [6] . The non-reciprocal metamaterial cell presented here is mechanically robust. The non-reciprocity is entirely implemented in electronics, which puts less stringent requirements on the physical materials composing the cell. It also allows tight control of the cell behaviour, and most importantly, highly subwavelength designs. Most useful acoustic applications are at frequencies below a couple of megahertz for which there are ubiquitous high-quality, high-speed commercial electronic components. In addition, the low propagation speed of acoustic waves means that the dynamic response of the device is almost simultaneous with the acoustic excitation, as demonstrated in this article. The design concept is based on metamaterial techniques and, as such, it is flexible in that it can be trivially modified to generate highly nonlinear reciprocal or non-reciprocal bulk media or arbitrary-shaped surfaces working at low frequencies and low sound levels in air or liquids. Moreover, this design method generates relatively broadband devices capable to preserve the envelope of the incident sound, which makes it a good candidate for numerous acoustic applications. How to cite this article: Popa, B.-I. and Cummer, S. A. Non-reciprocal and highly nonlinear active acoustic metamaterials. Nat. Commun. 5:3398 doi: 10.1038/ncomms4398 (2014).